Dietary sugar promotes systemic TOR activation inDrosophilathrough AKH-dependent selective secretion of Dilp3 Secreted ligands of the insulin family promote cell growth and maintain sugar homeostasis. Insulin release is tightly regulated in response to dietary conditions, but how insulin-producing cells (IPCs) coordinate their responses to distinct nutrient signals is unclear. Here we show that regulation of insulin secretion in Drosophila larvae has been segregated into distinct branches—whereas amino acids promote the secretion of Drosophila insulin-like peptide 2 (Dilp2), circulating sugars promote the selective release of Dilp3. Dilp3 is uniquely required for the sugar-mediated activation of TOR signalling and suppression of autophagy in the larval fat body. Sugar levels are not sensed directly by the IPCs, but rather by the adipokinetic hormone (AKH)-producing cells of the corpora cardiaca, and we demonstrate that AKH signalling is required in the IPCs for sugar-dependent Dilp3 release. Thus, IPCs integrate multiple cues to regulate the secretion of distinct insulin subtypes under varying nutrient conditions. Insulin signalling is a conserved mechanism regulating cell growth, differentiation and development. Under feeding conditions, insulin is secreted into the circulatory system and activates insulin receptors in peripheral cells [1] . Subsequent activation of downstream components of the insulin pathway such as phosphoinositide (PI) 3-kinase, AKT and target of rapamycin (TOR) leads to the uptake of nutrients and stimulation of protein and lipid synthesis. Insulin signalling also suppresses autophagy, a catabolic mechanism that produces an alternative source of nutrients through the degradation of cytoplasmic components [2] . This process involves the sequestration of cytoplasm within vesicular structures called autophagosomes, which fuse with lysosomes containing digestive enzymes. Induction of autophagy is inhibited by TOR, which in turn is activated both by insulin signalling and directly by intracellular nutrients, particularly amino acids. In addition to these effects on cell growth and autophagy, insulin also plays a well-characterized role in controlling the sugar levels in the blood. In mammals, pancreatic beta cells release insulin in response to high levels of glucose, leading to the uptake of glucose by other cells in the body to decrease sugar levels. When the level of glucose is low, pancreatic alpha cells secrete glucagon, a G protein-coupled receptor (GPCR) ligand that triggers glycogenolysis and gluconeogenesis to increase sugar levels. Basic mechanisms of insulin and glucagon signalling are conserved in Drosophila , which provides a useful animal model system to investigate the effects of these hormones on growth and metabolism [3] , [4] , [5] . Drosophila insulin-like peptides (Dilps) regulate cell growth and aging, and they maintain normal sugar levels in the haemolymph, the circulating fluid in insects. Eight Dilps have been identified, of which Dilp2, Dilp3 and Dilp5 are produced in the insulin-producing cells (IPCs) of the brain. Ablation of the IPCs causes hyperglycaemia in Drosophila larvae, and this phenotype can be rescued by ectopic expression of Dilp2 (ref. 6 ). In addition, the corpora cardiaca (CC) in the ring gland generate the GPCR ligand adipokinetic hormone (AKH), which has homologous functions to glucagon, contributing to sugar homeostasis as well as regulation of fat stores [7] , [8] . The secretion of Dilps from the IPCs is regulated by dietary nutrients through non-autonomous relay mechanisms. In response to dietary amino acids, the fat body produces an undefined signal that promotes Dilp2 secretion into the haemolymph [9] . In adult flies, the fat body secretes the JAK/STAT ligand Unpaired 2 in response to dietary nutrients, which also stimulates Dilp2 release [10] . Whether the secretion of other Dilps is controlled through similar mechanisms is unclear, and the direct effects of haemolymph sugar levels on Dilp release remain poorly understood. Here we show that Dilp2 and Dilp3 differ in their regulation by distinct classes of nutrients—whereas Dilp2 secretion responds selectively to amino acids, secretion of Dilp3 is stimulated primarily by glucose and trehalose, the major sugar present in Drosophila larval haemolymph. Further, we demonstrate that trehalose stimulates the CC to release AKH, which then acts directly on the IPCs to promote the secretion of Dilp3. Trehalose-mediated Dilp3 secretion from the IPCs leads to the upregulation of TOR signalling and suppression of autophagy in the larval fat body, and is required for sugar homeostasis and normal rates of larval development under nutritional stress. We propose that coupling AKH release to the selective secretion of Dilp3 plays a critical role in promoting sugar homeostasis under the conditions of high insulin signalling required for rapid cell growth during larval development. Trehalose promotes the activation of TOR in the larval fat body To examine how systemic insulin signalling activity is influenced by sugar levels in Drosophila larvae, we developed an ex vivo culture system in which dissected larval carcasses are incubated in medium with varying sugar concentrations. As a measure of insulin signalling in peripheral tissues, we first examined the activity of TOR in the larval fat body, a site of high sensitivity to insulin signalling. Incubation of inverted larval carcasses in M3 medium, a commonly used insect cell culture medium, led to a rapid decrease in TOR-dependent phosphorylation of S6K Thr398 in fat body extracts ( Fig. 1a ). We refer hereafter to this phosphorylation signal as fb-TOR activity. In contrast, fb-TOR activity was maintained when M3 medium was supplemented with glucose or trehalose, the two main sugars present in Drosophila haemolymph ( Fig. 1a , Supplementary Fig. 1a,b ). Sucrose, which is not a constituent of haemolymph, did not support fb-TOR activity ( Supplementary Fig. 1b ). As trehalose, but not glucose, promoted fb-TOR activity in the range of its normal physiological concentration in larval haemolymph [11] , we focused our further analysis on this disaccharide. 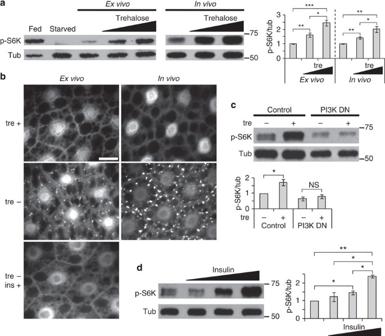Figure 1: Trehalose promotes TOR signalling in the larval fat body. (a) TOR activity was measured by immunoblot of wild-type fat body extracts with phospho-T398 S6K (p-S6K) antibody. Fed and starved controls (lanes 1 and 2) show the range of fb-TOR activity on standard fly food and following a 2-h starvation. In bothex vivo(larval carcasses incubated 2 h in M3 medium with 0, 20 or 40 mg ml−1trehalose) andin vivo(larvae cultured overnight in agar/tryptone food with 0, 13.3 or 26.6 mg ml−1trehalose) cultures, addition of trehalose (tre) results in a dose-dependent increase in p-S6K. Data represent mean±s.e.m. of four independent experiments. (b) Trehalose inhibits the formation of autophagic vesicles in larval fat body cells.Cg-Gal4/UAS-mCherry-Atg8acarcasses or larvae were incubated underex vivo(4 h in M3 medium ±20 mg ml−1trehalose) orin vivo(overnight on agar/tryptone food ±26.6 mg ml−1trehalose) conditions. Human insulin (ins, 10 μg ml−1) inhibits autophagosome formation inex vivocultures lacking trehalose. Scale bar, 20 μm. Images are representative of three experiments (seven larvae per condition). (c) PI 3-kinase activity is required forex vivoactivation of fb-TOR by trehalose. Expression of dominant negative p110 catalytic subunit in the fat body(Cg-GAL4/UAS-p110D954A) reduces fb-TOR activity and inhibits its response to trehalose. Data represent mean±s.e.m. of three independent experiments. (d) Addition of human insulin (0.01, 0.1 and 1 μg ml−1) toex vivocultures lacking trehalose causes dose-dependent increases in fb-TOR activity. Data represent mean±s.e.m. of three independent experiments. Graphs display ratios of p-S6K/tubulin (tub) band intensities, normalized to control. *P<0.05, **P<0.01, ***P<0.001, NS, not significant;P>0.05; Student’st-test. Full-size immunoblots are presented inSupplementary Fig. 4. Figure 1: Trehalose promotes TOR signalling in the larval fat body. ( a ) TOR activity was measured by immunoblot of wild-type fat body extracts with phospho-T398 S6K (p-S6K) antibody. Fed and starved controls (lanes 1 and 2) show the range of fb-TOR activity on standard fly food and following a 2-h starvation. In both ex vivo (larval carcasses incubated 2 h in M3 medium with 0, 20 or 40 mg ml −1 trehalose) and in vivo (larvae cultured overnight in agar/tryptone food with 0, 13.3 or 26.6 mg ml −1 trehalose) cultures, addition of trehalose (tre) results in a dose-dependent increase in p-S6K. Data represent mean±s.e.m. of four independent experiments. ( b ) Trehalose inhibits the formation of autophagic vesicles in larval fat body cells. Cg-Gal4/UAS-mCherry-Atg8a carcasses or larvae were incubated under ex vivo (4 h in M3 medium ±20 mg ml −1 trehalose) or in vivo (overnight on agar/tryptone food ±26.6 mg ml −1 trehalose) conditions. Human insulin (ins, 10 μg ml −1 ) inhibits autophagosome formation in ex vivo cultures lacking trehalose. Scale bar, 20 μm. Images are representative of three experiments (seven larvae per condition). ( c ) PI 3-kinase activity is required for ex vivo activation of fb-TOR by trehalose. Expression of dominant negative p110 catalytic subunit in the fat body (Cg-GAL4/UAS-p110 D954A ) reduces fb-TOR activity and inhibits its response to trehalose. Data represent mean±s.e.m. of three independent experiments. ( d ) Addition of human insulin (0.01, 0.1 and 1 μg ml −1 ) to ex vivo cultures lacking trehalose causes dose-dependent increases in fb-TOR activity. Data represent mean±s.e.m. of three independent experiments. Graphs display ratios of p-S6K/tubulin (tub) band intensities, normalized to control. * P <0.05, ** P <0.01, *** P <0.001, NS, not significant; P >0.05; Student’s t- test. Full-size immunoblots are presented in Supplementary Fig. 4 . Full size image The effects of trehalose ex vivo were recapitulated in in vivo feeding experiments. Larvae raised on agar/tryptone food containing trehalose showed dose-dependent activation of TOR in the fat body compared with food lacking trehalose ( Fig. 1a ). As a physiological readout of this pathway, we monitored the effect of trehalose on the induction of autophagy, which is inhibited by TOR signalling. Both in vivo feeding and ex vivo incubation in the absence of trehalose led to the formation of mCherry-Atg8-positive autophagosomes and autolysosomes throughout the larval fat body within 4 h. Inclusion of trehalose in these experiments prevented autophagy induction ( Fig. 1b ). Ex vivo incubation in a more severe starvation medium (EBSS supplemented with leucine) also led to autophagy induction that was suppressed by trehalose ( Supplementary Fig. 1c ). Together these data suggest that both dietary and circulating haemolymph trehalose can promote TOR activation in the larval fat body. Trehalose regulates systemic insulin signalling Several lines of evidence indicated that activation of TOR by trehalose may be mediated by insulin signalling. First, trehalose-dependent TOR activation was strongly inhibited by expression in the fat body of a dominant negative subunit of PI 3-kinase, a central component of the insulin pathway ( Fig. 1c ). Second, the ex vivo requirement for trehalose to maintain fb-TOR activation and suppress autophagy was bypassed by the inclusion of human insulin in the medium ( Fig. 1b,d ). Finally, trehalose promoted the phosphorylation of Akt on Ser505, a site of activation regulated by insulin signalling ( Supplementary Fig. 1d ). Of the eight Drosophila insulin-like proteins, Dilp2, Dilp3 and Dilp5 are expressed in twin clusters of IPCs within the central nervous system (CNS). To examine the potential involvement of these brain-derived Dilps in mediating the systemic effects of trehalose, we first tested whether the CNS itself is required for trehalose-stimulated activation of TOR. Whereas trehalose promoted the dose-dependent S6K phosphorylation in the fat body of complete carcasses, removal of the brain and associated ring gland complex abrogated this response ( Fig. 2a ). Trehalose also failed to suppress autophagy induction in the fat body of brain-less larval carcasses ( Fig. 2b ). To ask whether soluble factors from the brain are released into the media, we pretreated M3+trehalose medium by incubation with larval brain/ring gland complexes. This conditioned medium was able to fully activate S6K phosphorylation in the fat body of brain-less carcasses ( Fig. 2c ). In contrast, the medium conditioned with CNS complexes from larvae mutant for Dilps1–5 and Dilp7 was significantly less effective in this assay. These results indicate that trehalose-dependent activation of TOR in the larval fat body is a non-autonomous response requiring a CNS-derived signal, and that one or more of the brain-derived Dilps are required for a significant portion of this signal. 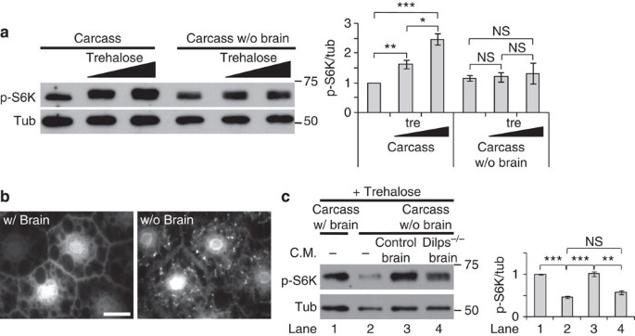Figure 2: Trehalose-dependent activation of TOR in the larval fat body requires the brain and insulin signalling. (a) Supplementation of M3 medium with trehalose (0, 20, 40 mg ml−1) leads to significant increases in fb-TOR activity from whole-larval carcasses (left) but not in carcasses from which the brain was surgically removed (right). Data represent mean±s.e.m. of four independent experiments. (b) Trehalose (20 mg ml−1in M3) suppresses the formation of autophagic vesicles (mCherry-Atg8 punctae) in fat body cells of complete carcasses but not carcasses lacking the brain. Scale bar, 20 μm. Representative images of three experiments (seven carcasses per condition). (c) Fb-TOR activity of carcasses lacking the brain, incubated in control M3+trehalose medium (−), or in M3+trehalose conditioned medium (C.M.) previously incubated 2 h with CNS complexes from wild-type larvae (control brain) or from mutant larvae lackingDilps1–5andDilp7(Dilps−/−brain). Data represent mean±s.e.m. of four independent experiments. *P<0.05, **P<0.01, ***P<0.001, NS, not significant;P>0.05; Student’st-test. Full-size immunoblots are shown inSupplementary Fig. 4. Figure 2: Trehalose-dependent activation of TOR in the larval fat body requires the brain and insulin signalling. ( a ) Supplementation of M3 medium with trehalose (0, 20, 40 mg ml −1 ) leads to significant increases in fb-TOR activity from whole-larval carcasses (left) but not in carcasses from which the brain was surgically removed (right). Data represent mean±s.e.m. of four independent experiments. ( b ) Trehalose (20 mg ml −1 in M3) suppresses the formation of autophagic vesicles (mCherry-Atg8 punctae) in fat body cells of complete carcasses but not carcasses lacking the brain. Scale bar, 20 μm. Representative images of three experiments (seven carcasses per condition). ( c ) Fb-TOR activity of carcasses lacking the brain, incubated in control M3+trehalose medium (−), or in M3+trehalose conditioned medium (C.M.) previously incubated 2 h with CNS complexes from wild-type larvae (control brain) or from mutant larvae lacking Dilps1–5 and Dilp7 (Dilps −/− brain). Data represent mean±s.e.m. of four independent experiments. * P <0.05, ** P <0.01, *** P <0.001, NS, not significant; P >0.05; Student’s t -test. Full-size immunoblots are shown in Supplementary Fig. 4 . Full size image Trehalose activates TOR via selective secretion of Dilp3 The requirement for the CNS implicates Dilp2, Dilp3 and/or Dilp5 in trehalose-responsive signalling. To directly test the potential role of these factors, we examined the effects of trehalose in mutant animals individually lacking each Dilp. Whereas homozygous Dilp2 and Dilp5 mutants each showed normal fat body TOR activation following ex vivo incubation in trehalose-containing media, this response was defective in Dilp3 mutant larvae ( Fig. 3a ). Similarly, mutation of Dilp3 but not Dilp2 or Dilp5 strongly reduced fb-TOR signalling in vivo in response to inclusion of trehalose in the diet ( Fig. 3b ). Thus, we conclude that trehalose elicits systemic insulin signalling primarily through Dilp3. 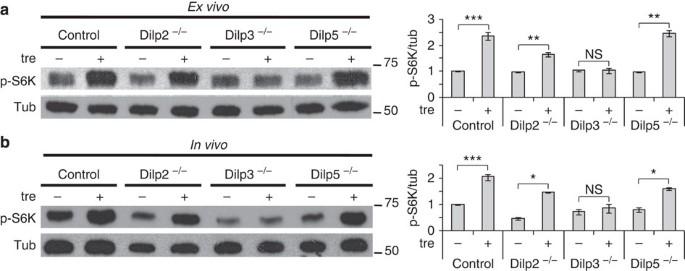Figure 3: Dilp3 is required for TOR activation by trehalose. (a)Ex vivoincubation of larval carcasses in M3 medium supplemented with or without 40 mg ml−1trehalose. Trehalose promotes fb-TOR activity in control,Dilp2−/−andDilp5−/−larvae, but not inDilp3−/−larvae. (b)In vivoincubation of larvae in agar/tryptone food containing 0 or 26.6 mg ml−1trehalose. Fb-TOR activity is significantly increased by trehalose in control,Dilp2−/−andDilp5−/−larvae, but not inDilp3−/−larvae. Representative blots of three independent experiments are shown in each panel. Data were assessed by Student’st-test and are represented as mean±s.d. *P<0.05, **P<0.01, ***P<0.001, NS, not significant;P>0.05. Full-size immunoblots are presented inSupplementary Fig. 5. Figure 3: Dilp3 is required for TOR activation by trehalose. ( a ) Ex vivo incubation of larval carcasses in M3 medium supplemented with or without 40 mg ml −1 trehalose. Trehalose promotes fb-TOR activity in control, Dilp2 −/− and Dilp5 −/− larvae, but not in Dilp3 −/− larvae. ( b ) In vivo incubation of larvae in agar/tryptone food containing 0 or 26.6 mg ml −1 trehalose. Fb-TOR activity is significantly increased by trehalose in control, Dilp2 −/− and Dilp5 −/− larvae, but not in Dilp3 −/− larvae. Representative blots of three independent experiments are shown in each panel. Data were assessed by Student’s t- test and are represented as mean±s.d. * P <0.05, ** P <0.01, *** P <0.001, NS, not significant; P >0.05. Full-size immunoblots are presented in Supplementary Fig. 5 . Full size image Géminard et al. [9] showed previously that dietary amino acids promote the secretion of Dilp2 from the IPCs, and that Dilp2 protein accumulates to high levels in these cells in response to amino-acid starvation. We used a similar immunostaining approach to examine the effects of trehalose on Dilp accumulation and release. Following ex vivo incubation in M3 medium supplemented with trehalose, protein levels of both Dilp2 and Dilp3 were low in the IPCs, as assayed by antibodies specific for either Dilp2 or Dilp3 (see Supplementary Fig. 2a,b for antibody-control experiments). In contrast, incubation in the medium lacking trehalose led to a marked accumulation of Dilp3, but not Dilp2, in these cells ( Fig. 4a ). Similar effects were observed in vivo —staining intensity of both Dilps was low in the IPCs of larvae raised on food rich in amino acids and trehalose, and removal of trehalose from the diet led to accumulation of Dilp3 but not Dilp2 ( Fig. 4b ). Starvation for amino acids had the opposite effect, increasing the intensity of Dilp2 staining, as reported, but not that of Dilp3. The expression of Dilp2 and Dilp3 mRNA was unchanged in response to these dietary conditions ( Fig. 4c ). Finally, the larvae raised on food containing trehalose had a higher level of circulating Dilp3 protein in the haemolymph ( Fig. 4d ), consistent with the low Dilp3 levels in the IPCs under these conditions. Thus, whereas the mRNA levels of both Dilp2 and 3 have been shown to increase in response to a high-sugar diet and to correlate with glucose and trehalose haemolymph concentrations [12] , our data indicate that only Dilp3 is regulated by sugar at the level of secretion. Taken together, we conclude that the secretion of Dilp2 and Dilp3 is independently regulated by amino acids and trehalose, respectively. 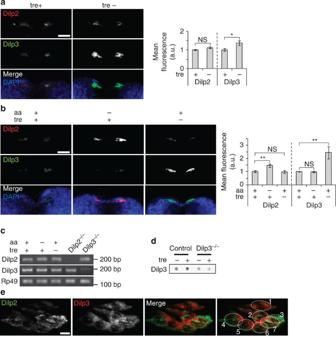Figure 4: Trehalose promotes the secretion of Dilp3. (a) Confocal images showing Dilp2 and Dilp3 proteins followingex vivoincubation in the presence or absence of trehalose. Incubation in the medium lacking trehalose leads to Dilp3 accumulation in the IPCs, whereas Dilp2 staining remains low under both conditions. (b) Accumulation of Dilp2 and Dilp3 in response toin vivostarvation for amino acids (aa) or trehalose. Levels of Dilp2 and Dilp3 are low in the IPCs of larvae raised on agar/tryptone/trehalose food. Dilp2 accumulates in response to lack of dietary amino acids (tryptone) but not trehalose, whereas Dilp3 accumulates in larvae raised on food lacking trehalose but not amino acids. Images ina,bare representative of eight larvae. Data were assessed by Student’st-test and are represented as mean±s.d. *P<0.05, **P<0.01, NS, not significant;P>0.05. a.u., arbitrary units. (c) Levels ofDilp2andDilp3mRNA in response toin vivostarvation for amino acids or trehalose, analysed by semi-quantitative reverse transcription–PCR.Rp49serves as internal control. Representative results of three independent experiments are shown. (d) Dot blot analysis of circulating Dilp3 levels in larvae grown on food with or without trehalosein vivo. Blot is representative of three independent experiments. (e) High-magnification combinedZ-series stack of confocal sections of IPCs from 24 h starved larvae, demonstrating distinct intracellular localization and biased expression of Dilp2 and Dilp3. Image is representative of three experiments,n=7 larvae. Scale bars , 50 μm ina,band 5 μm ine. Full-sized gel and dot blot scans are presented inSupplementary Fig. 5. Figure 4: Trehalose promotes the secretion of Dilp3. ( a ) Confocal images showing Dilp2 and Dilp3 proteins following ex vivo incubation in the presence or absence of trehalose. Incubation in the medium lacking trehalose leads to Dilp3 accumulation in the IPCs, whereas Dilp2 staining remains low under both conditions. ( b ) Accumulation of Dilp2 and Dilp3 in response to in vivo starvation for amino acids (aa) or trehalose. Levels of Dilp2 and Dilp3 are low in the IPCs of larvae raised on agar/tryptone/trehalose food. Dilp2 accumulates in response to lack of dietary amino acids (tryptone) but not trehalose, whereas Dilp3 accumulates in larvae raised on food lacking trehalose but not amino acids. Images in a , b are representative of eight larvae. Data were assessed by Student’s t- test and are represented as mean±s.d. * P <0.05, ** P <0.01, NS, not significant; P >0.05. a.u., arbitrary units. ( c ) Levels of Dilp2 and Dilp3 mRNA in response to in vivo starvation for amino acids or trehalose, analysed by semi-quantitative reverse transcription–PCR. Rp49 serves as internal control. Representative results of three independent experiments are shown. ( d ) Dot blot analysis of circulating Dilp3 levels in larvae grown on food with or without trehalose in vivo . Blot is representative of three independent experiments. ( e ) High-magnification combined Z -series stack of confocal sections of IPCs from 24 h starved larvae, demonstrating distinct intracellular localization and biased expression of Dilp2 and Dilp3. Image is representative of three experiments, n =7 larvae. Scale bars , 50 μm in a , b and 5 μm in e . Full-sized gel and dot blot scans are presented in Supplementary Fig. 5 . Full size image How might different nutrient cues promote the selective secretion of distinct insulin-like peptides? Individual secretion granules containing Dilps can be visualized within the IPCs by high-powered confocal imaging. Analysis of brains double-labelled for Dilp2 and Dilp3 revealed that while some of these granules contain both Dilps, many contain largely either Dilp2 or Dilp3 ( Fig. 4e , Supplementary Fig. 2c,d ). Interestingly, granules containing Dilp2 or Dilp3 tend to segregate to distinct regions of the cell. In addition, many individual IPCs show a clear bias in the levels of one Dilp over another. Thus, the activation of distinct release pathways and/or subclasses of IPCs may contribute to these nutrient-selective responses. An AKH-Dilp3 relay mediates trehalose-dependent TOR signalling In mammals, ATP-sensitive potassium channels in the pancreatic beta cells play a critical role in sensing glucose levels and regulating insulin secretion. Interestingly, Drosophila homologues of these channel subunits are absent from larval IPCs, but instead are specifically expressed in the CC cells of the ring gland [7] . These cells express the glucagon-like hormone AKH, and they make contact with processes from the IPCs. We found that RNA interference (RNAi)-mediated depletion of AKH in the CC, or ablation of the CC itself, inhibited fat body TOR activation in response to trehalose ( Fig. 5a ; see Supplementary Fig. 3a for depletion and ablation controls). Null mutation of the AKH receptor ( AKHR ) showed a similar block in TOR activation ( Fig. 5b ). Conversely, the overexpression of AKH increased TOR activity in both the presence and absence of trehalose ( Fig. 5c ). 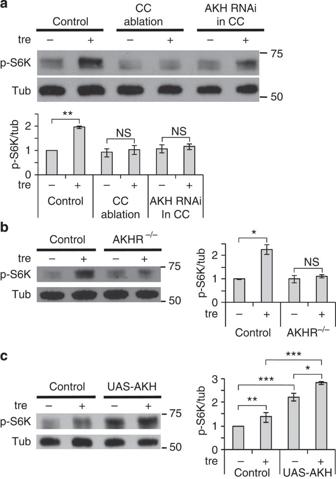Figure 5: Activation of TOR by trehalose requires AKH signalling. (a,b) Trehalose-mediatedex vivoactivation of fb-TOR is disrupted by ablation of the CC(AKH-GAL4/UAS-reaper)or depletion ofAKHfrom the CC(AKH-GAL4/UAS-AKHRNAi) and by null mutation of the AKH receptor(AKHR1/AKHR1). (c) Overexpression of AKH(Cg-GAL4/UAS-Akh)increases fb-TOR signalling in the presence and absence of trehaloseex vivo. Data represent mean±s.e.m. of three (a,b) or four (c) independent experiments. *P<0.05, **P<0.01, ***P<0.001, NS, not significant;P>0.05; Student’st-test. Full-sized immunoblots are presented inSupplementary Fig. 5. Figure 5: Activation of TOR by trehalose requires AKH signalling. ( a , b ) Trehalose-mediated ex vivo activation of fb-TOR is disrupted by ablation of the CC (AKH-GAL4/UAS-reaper) or depletion of AKH from the CC (AKH-GAL4/UAS-AKH RNAi ) and by null mutation of the AKH receptor (AKHR 1 /AKHR 1 ). ( c ) Overexpression of AKH (Cg-GAL4/UAS-Akh) increases fb-TOR signalling in the presence and absence of trehalose ex vivo . Data represent mean±s.e.m. of three ( a , b ) or four ( c ) independent experiments. * P <0.05, ** P <0.01, *** P <0.001, NS, not significant; P >0.05; Student’s t- test. Full-sized immunoblots are presented in Supplementary Fig. 5 . Full size image The influence of AKH signalling on trehalose-dependent TOR activation suggested that the secretion of AKH may be regulated by trehalose. Although previous studies using fluorescent calcium sensors indicate that the acute reduction in trehalose may stimulate secretion from CC cells [7] , [13] , AKH protein levels in the CC were markedly increased following a 2-h incubation in the medium lacking trehalose ( Fig. 6a ). This accumulation of AKH can be attributed to decreased secretion rather than increased production, as cycloheximide was included in these experiments to inhibit the synthesis of new protein. Furthermore, the CC-specific expression of the exocytosis inhibitor tetanus toxin, which has been shown to inhibit AKH secretion [13] , prevented the reduction in AKH staining in response to trehalose ( Fig. 6a ). To confirm that the release and diffusion of AKH is required for TOR activation in the fat body, we depleted AKH from the medium by adding a blocking antibody against AKH, which led to a dose-dependent decrease in the trehalose-stimulated fb-TOR activity ( Fig. 6b ). Altogether, these results indicate that the secretion of AKH from the CC is an essential intermediary step in trehalose-responsive TOR activation. 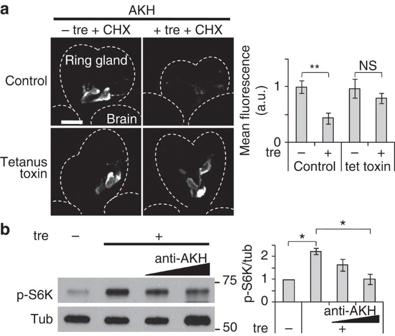Figure 6: Trehalose promotes AKH secretion to stimulate fb-TOR signalling. (a) AKH antibody staining in the CC is reduced in response to trehalose duringex vivoincubation. CC-specific expression of tetanus toxin(AKH-GAL4/UAS-TeTxLC)prevents the effect of trehalose. Cycloheximide (25 μg ml−1) was included in all incubations to block AKH synthesis. Scale bar, 50 μm. Representative images of seven ring glands per experimental condition are shown. (b)Ex vivoactivation of fb-TOR signalling in response to trehalose is inhibited by blocking antibody against AKH (2 × 10−3and 4 × 10−3serum dilution in M3 media). Blot is representative of three independent experiments. Bar graphs ina,brepresent mean±s.e.m. *P<0.05, **P<0.01, NS, not significant;P>0.05; Student’st-test. Full-sized immunoblots are shown inSupplementary Fig. 6. Figure 6: Trehalose promotes AKH secretion to stimulate fb-TOR signalling. ( a ) AKH antibody staining in the CC is reduced in response to trehalose during ex vivo incubation. CC-specific expression of tetanus toxin (AKH-GAL4/UAS-TeTxLC) prevents the effect of trehalose. Cycloheximide (25 μg ml −1 ) was included in all incubations to block AKH synthesis. Scale bar, 50 μm. Representative images of seven ring glands per experimental condition are shown. ( b ) Ex vivo activation of fb-TOR signalling in response to trehalose is inhibited by blocking antibody against AKH (2 × 10 −3 and 4 × 10 −3 serum dilution in M3 media). Blot is representative of three independent experiments. Bar graphs in a , b represent mean±s.e.m. * P <0.05, ** P <0.01, NS, not significant; P >0.05; Student’s t- test. Full-sized immunoblots are shown in Supplementary Fig. 6 . Full size image The similar effects of AKH and Dilp3 are consistent with these factors acting in a common pathway to communicate trehalose levels to peripheral tissues. We therefore asked whether AKH signalling is required in the IPCs for fb-TOR activity. Indeed, IPC-specific knockdown of AKHR significantly inhibited the activation of TOR in the fat body in response to trehalose ( Fig. 7a ). These results support the possibility that AKH signalling in the IPCs may be necessary for the trehalose-stimulated release of Dilp3. Consistent with this hypothesis, Dilp3 protein accumulated to high levels in the IPCs in response to depletion of AKH in the CC, in AKH receptor null mutants, and in response to depletion of AKHR specifically in the IPCs ( Fig. 7b ). These manipulations had no effect on Dilp3 mRNA levels ( Fig. 7c ). We conclude that the IPCs are important targets of AKH signalling, releasing Dilp3 in response to a trehalose-AKH relay from the CC cells. 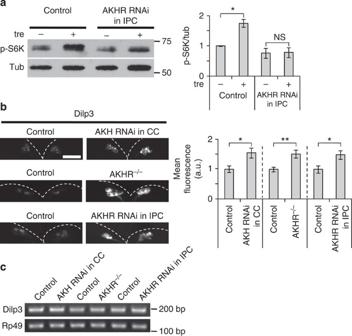Figure 7: AKH signalling in the IPCs is required for Dilp3 release. (a) Depletion ofAKHRby RNAi in the IPCs(Dilp2-GAL4/UAS-AKHRRNAi) impairs TOR activation in the fat body in response to trehalose in the media. Blot is representative of three independent experiments. (b) Followingex vivoincubation in the presence of trehalose, Dilp3 protein accumulates in the IPCs in response to depletion ofAKHin the CC(AKH-GAL4/UAS-AKHRNAi), null mutation ofAKHR (AKHR1/Df (2L)Exel7027)and depletion ofAHKRin the IPCs(Dilp2-GAL4/UAS-AKHRRNAi). Scale bar, 50 μm. Representative images of eight animals per genotype are shown. Data ina,bwere assessed by Student’st-test and are represented as mean±s.d. *P<0.05, **P<0.01, NS, not significant;P>0.05. (c) Levels ofDilp3mRNA in the genotypes indicated inb, analysed by semi-quantitative reverse transcription–PCR.Rp49serves as internal control. Blot is representative of three independent experiments. Full-sized immunoblots and gels are presented inSupplementary Fig. 6. Figure 7: AKH signalling in the IPCs is required for Dilp3 release. ( a ) Depletion of AKHR by RNAi in the IPCs (Dilp2-GAL4/UAS-AKHR RNAi ) impairs TOR activation in the fat body in response to trehalose in the media. Blot is representative of three independent experiments. ( b ) Following ex vivo incubation in the presence of trehalose, Dilp3 protein accumulates in the IPCs in response to depletion of AKH in the CC (AKH-GAL4/UAS-AKH RNAi ), null mutation of AKHR (AKHR 1 /Df (2L)Exel7027) and depletion of AHKR in the IPCs (Dilp2-GAL4/UAS-AKHR RNAi ). Scale bar, 50 μm. Representative images of eight animals per genotype are shown. Data in a , b were assessed by Student’s t -test and are represented as mean±s.d. * P <0.05, ** P <0.01, NS, not significant; P >0.05. ( c ) Levels of Dilp3 mRNA in the genotypes indicated in b , analysed by semi-quantitative reverse transcription–PCR. Rp49 serves as internal control. Blot is representative of three independent experiments. Full-sized immunoblots and gels are presented in Supplementary Fig. 6 . Full size image Dilp3 effects developmental rate and sugar homeostasis Although insulin signalling is essential for normal growth and development, mutation of most individual Dilps has surprisingly little developmental effect, presumably due to redundancy and compensation between these factors [14] , [15] . In particular, mutants lacking Dilp3 develop with normal timing and show only a modest reduction in fecundity. We confirmed this lack of effect on the developmental rate when Dilp3 mutant and control animals were raised on rich medium supplemented with yeast. However, growth on the medium lacking yeast resulted in a 30-h delay in development in Dilp3 mutant compared with control animals ( Fig. 8a ). These results reveal a cryptic growth requirement for Dilp3, presumably made evident here due to the reduced levels of Dilp2 and/or Dilp5 under conditions of low amino acids. Interestingly, AKHR mutants showed a similarly enhanced developmental delay in the absence of dietary yeast ( Supplementary Fig. 3b ), further supporting that AKH and Dilp3 function in a common pathway. In addition, the levels of circulating trehalose were significantly higher in Dilp3 mutant larvae than controls, particularly under the fed conditions required for Dilp3 release ( Fig. 8b , Supplementary Fig. 3c ). Altogether, these results are consistent with a central role for Dilp3 in mediating growth and metabolism in response to dietary sugar. 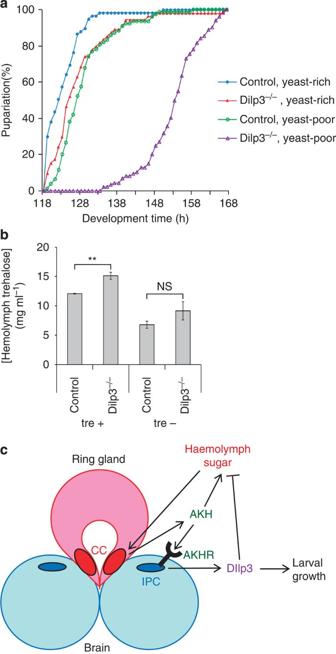Figure 8: Dilp3 affects larval growth and sugar homeostasis. (a) Developmental timing from egg laying to pupariation of control andDilp3−/−mutants raised on rich and poor medium (standard fly food with and without supplementary yeast, respectively). Data are from three vials of 30 larvae for each experimental condition. (b) Levels of circulating trehalose in control andDilp3−/−larvae cultured in the presence or absence of trehalosein vivo. Data of three independent experiments were assessed by Student’st-test and are represented as mean±s.d. **P<0.01, NS, not significant;P>0.05. (c) The results are consistent with a model whereby sugar stimulates the release of AKH from the CC, which then triggers the secretion of Dilp3 from the IPCs. Increased insulin signalling in peripheral tissues promotes larval growth, sugar uptake and activation of TOR in the fat body, the latter of which may lead to further signal amplification through subsequent stimulation of Dilp2 release from the IPCs. The sugar-dependent secretion of AKH represents another potential positive feedback loop, which may be restricted by the counterbalancing effect of Dilp3. This model implies that in rapidly growingDrosophilalarvae, co-regulation of AKH and insulin signalling may support high rates of insulin-dependent anabolic growth while preventing excessive storage of trehalose in the fat body, allowing other cells to use sugar to fuel cell growth. Figure 8: Dilp3 affects larval growth and sugar homeostasis. ( a ) Developmental timing from egg laying to pupariation of control and Dilp3 −/− mutants raised on rich and poor medium (standard fly food with and without supplementary yeast, respectively). Data are from three vials of 30 larvae for each experimental condition. ( b ) Levels of circulating trehalose in control and Dilp3 −/− larvae cultured in the presence or absence of trehalose in vivo . Data of three independent experiments were assessed by Student’s t- test and are represented as mean±s.d. ** P <0.01, NS, not significant; P >0.05. ( c ) The results are consistent with a model whereby sugar stimulates the release of AKH from the CC, which then triggers the secretion of Dilp3 from the IPCs. Increased insulin signalling in peripheral tissues promotes larval growth, sugar uptake and activation of TOR in the fat body, the latter of which may lead to further signal amplification through subsequent stimulation of Dilp2 release from the IPCs. The sugar-dependent secretion of AKH represents another potential positive feedback loop, which may be restricted by the counterbalancing effect of Dilp3. This model implies that in rapidly growing Drosophila larvae, co-regulation of AKH and insulin signalling may support high rates of insulin-dependent anabolic growth while preventing excessive storage of trehalose in the fat body, allowing other cells to use sugar to fuel cell growth. Full size image The dual roles of insulin in promoting both cell growth and sugar homeostasis impose a unique challenge during periods of high growth such as larval and fetal development—sustained insulin signalling is required for normal developmental growth, yet circulating sugar concentrations must be maintained at a steady level under varying nutritional conditions. The results presented here suggest that in Drosophila larvae, this challenge is met in part through the coupled secretion of Dilp3 and AKH ( Fig. 8c ). This allows for normal haemolymph sugar concentrations despite relatively high Dilp levels, due to the counteracting effects of AKH. Although these hormones have opposing effects on haemolymph sugar concentrations akin to those of mammalian insulin and glucagon, their mechanisms of action are distinct. Ablation of the IPCs or deletion of Dilps 1–5 leads to increased haemolymph sugar concentrations [6] , [14] , likely reflecting a conserved role of Dilps in promoting glucose utilization and uptake through trafficking of glucose transporters [16] . In contrast, the manipulation of AKH signalling, through CC ablation or AKH overexpression, strongly effects the concentration of trehalose, but has little or no effect on glucose levels [8] . This hypertrehalosemic effect of AKH is widely conserved in insects, and reflects the unique features of trehalose as both a circulating and storage form of carbohydrate. Owing to the non-reactive, non-reducing properties of trehalose, its concentration can vary over a much wider range than glucose without causing cellular damage [17] . Haemolymph trehalose concentrations are commonly more than 10-fold higher than those of glucose, presumably due to the rapid conversion of glucose to trehalose in the fat body by trehalose-6-phosphate synthase [18] . This may counteract the low efficiency of insect open circulatory systems, bringing high concentrations of trehalose directly to cells, each molecule of which can be cleaved within the cell to provide two glucose molecules as needed. Thus, the effect of AKH on trehalose and total sugar levels likely masks smaller changes in glucose concentrations that may be more directly regulated by Dilps. Finally, in contrast to their opposing effects on sugar homeostasis, it is notable that AKH and insulin signalling act in the same direction to promote the expression of the α-glucosidase gene target of brain insulin (tobi) [19] . Together with the stimulation of Dilp3 secretion by AKH described here, these findings indicate that in addition to its glucagon-like role, AKH may also function as a homologue to glucagon-like peptide-1, a positive regulator of mammalian insulin signalling [20] . In contrast to the effect of trehalose as an autophagy suppressor described here, trehalose has been shown to activate autophagy in cultured mammalian cells, through undefined mechanisms [21] . Recently, Inoue and coworkers [22] demonstrated that sugars such as trehalose, sucrose and raffinose that cannot be hydrolysed by mammalian cells induce autophagy, whereas cleavable disaccharides such as maltose and fructose do not. In this regard, it is notable that both the larval fat body and the CC cells express trehalase, which catalyses the conversion of trehalose to glucose [7] . Indeed, it is unclear whether trehalose might be directly sensed and imported by the CC, or first converted to glucose through trehalases expressed on the cell surface [17] . The division of labour between Dilp2 and Dilp3 in responding to amino acids and sugars likely contributes to the ability of insulin signalling to balance the growth and metabolic requirements, allowing overall insulin signalling to remain high in growing larvae, while individual Dilps fluctuate in response to specific changes in nutrient conditions. This view implies that each of the eight Dilps may have evolved unique physiological functions in line with their specific mode of regulation. Whether different Dilps are functionally distinct remains poorly understood, but key differences between Dilp2 and Dilp3 may make them uniquely suited for growth and sugar homeostasis, respectively. For example, Dilp2 has been shown to have the strongest growth-promoting properties of Dilps1–7 when overexpressed during larval development [23] . Notably, the insulin-binding factors Imp-L2 and dALS are able to form protein complexes with Dilp2 but not Dilp3, whereas Dilp3 but not Dilp2 interacts strongly with the insulin receptor decoy SDR [24] , [25] , suggesting that individual Dilps may engage the insulin receptor in qualitatively different ways. Interestingly, the expression of Dilp5 is upregulated in dilp2 mutants and downregulated in dilp3 mutants [15] , indicating that these factors can have different and even opposing cellular effects, despite utilizing the same insulin receptor. Finally, recent studies have shown that selective outputs of insulin signalling can show distinct responses to transient versus sustained patterns of receptor activation [26] . In this regard, we note that although we show here that Dilp3, but not Dilp2, is involved in acute responses to altered sugar levels, a chronic high-sugar diet can increase the circulating levels of overexpressed Dilp2 (refs 12 , 27 ), and mutation of dilp2 leads to increased haemolymph trehalose levels by adulthood [15] . As the secretion of Dilp2 is promoted by activation of TOR in the fat body [9] , our finding that Dilp3 mediates fb-TOR activation by trehalose suggests that acute and chronic responses to sugar may be linked by a feed-forward mechanism, whereby the initial secretion of Dilp3 promotes subsequent Dilp2 secretion and further amplification of insulin signalling. The selective secretion of Dilp2 and Dilp3 in response to distinct nutritional cues suggests that Dilp peptides contain unique sequence or structural cues targeting them to distinct secretory pathways, or that homophilic interactions promotes self-sorting of these peptides. Indeed, confocal analysis revealed the clear segregation of Dilp2 and Dilp3 into different granules and intracellular regions. Selective secretion in response to a number of distinct stimuli has been described in eosinophils and mast cells—through a process known as piecemeal degranulation, specific cytokines are sequestered from secretion granules and shuttled to the plasma membrane in distinct secretory vesicles [28] . This sequestration step involves direct ligand–receptor interaction within secretory pathway compartments. Similarly, the release of specific classes of neurotransmitters from individual nerve terminals can be differentially stimulated in response to varying levels of Ca 2+ concentration [29] . In mouse islet beta cells, glucagon-like peptide-1 was recently shown to selectively promote the secretion of newly synthesized secretory granules over that of granules previously docked at the plasma membrane [30] . As the three receptors shown to regulate Dilp secretion—GABA-R [10] , adiponectinR [31] and AKHR (present study)—are each members of the GPCR family, it will be interesting to investigate how the different modes of downstream signalling ultimately affect selective Dilp release. Drosophila strains The following D. melanogaster strains were used: AKHR[1] , AKHR[revA] (ref. 32 , gift of R. Kühnlein, Max Planck Institute, Göttingen, Germany); AKH[KK105063] and AKHR[KK109300] RNAi lines (Vienna Drosophila RNAi Center, Vienna, Austria); UAS-mChAtg8a (ref. 33 ); Akh-GAL4.L, Cg-GAL4.A, Df(2L)Exel7027, Dilp2-Gal4.R, Dilp2[1] , Dilp3[1], Dilp5[1], Df(3L)Dilp1-4 Dilp5[4] Dilp7[1], Oregon-R-C, UAS-Akh.L, UAS-Dp110[D954A], UAS-rpr.C, and UAS-TeTxLC. (−)Q were obtained from the Bloomington Drosophila Stock Center (Bloomington, IN). Larval culture Embryos were collected for 3–5 h on standard fly food. For in vivo feeding experiments, early L3 larvae (85–90 h after egg laying at 25 °C) were transferred to agar/tryptone medium containing 5.76 mg ml −1 of agar, 17 mg ml −1 of tryptone, 2 mg ml −1 of leucine with or without 26.6 mg ml −1 of trehalose for 15–17 h before dissection. For ex vivo carcass incubation experiments, L3 larvae (72–77 h after egg laying) were transferred to fresh standard fly food supplemented with granular yeast. After 24 h, seven larvae per condition were bisected and inverted and digestive tracks removed. Dissected carcasses were incubated with nutation at room temperature in 1 ml of Shields and Sang M3 Insect Medium (not serum supplemented) with or without trehalose (40 mg ml −1 or otherwise noted) for 2 h (for western blotting) or 4 h (autophagy experiments). M3 medium (S3652), trehalose (T0167), human insulin solution (I9278), Earle’s Balanced Salts Solution (E3024) and L -Leucine (L8000) were from Sigma-Aldrich (St Louis, MO). Conditioned medium was made by incubating brain and ring gland complexes from 10 larvae for 2 h in 1 ml of M3 medium containing 40 mg ml −1 trehalose. The recovered medium was used immediately for incubation with carcasses from which the brain was removed. Immunoblotting Fat bodies from five larvae per sample were dissected in PBS and lysed directly in SDS sample buffer, with three or more biological replicates used for each experiment. Extracts were boiled 3 min, separated by polyacrylamide gel electrophoresis and transferred to Immobilon-P membranes (Millipore, Billerica MA). Circulating Dilp3 levels were determined from haemolymph of 10 larvae per sample, diluted 1:100 in PBS and spotted (1 μl) onto methanol-soaked Immobilon-P membranes (Millipore, Billerica MA). Air-dried membranes were blocked in PBS+0.1% Tween20+5% bovine serum albumin, and incubated overnight in blocking solution containing primary antibody. Signals were visualized using SuperSignal West Pico chemiluminescent substrate (Thermo Scientific, Rockford, IL) with BioMax Light (Kodak, Rochester NY) or HyBlot CL autoradiography film (Denville Scientific, Metuchen NJ) and quantitated using Adobe Photoshop software. Antibodies used were rabbit anti-phospho-T398 dS6K (1:250), rabbit anti-phospho-S505 dAkt (1:1,000), (both from Cell Signaling Technology, Beverly MA), rabbit anti-Dilp3 (1:1,000; gift of J. Veenstra, Université Bordeaux, Talence, France [34] ) and mouse anti-beta-tubulin E7 (1:1,000; Developmental Studies Hybridoma Bank, Iowa City IA). Confocal imaging Samples were prepared for confocal imaging as follows—7–10 larvae were bisected and inverted in PBS, fixed 20 min in 4% paraformaldehyde/PBS, washed extensively in PBS+Triton-X-100 (PBT; 0.3 or 0.1% for imaging IPCs or CCs, respectively), blocked in PBT+5% bovine serum albumin and incubated overnight in blocking solution containing primary antibody. After four washes in PBT, samples were incubated for 2 h in blocking solution containing secondary antibody and washed four times. Carcasses after incubation ex vivo were directly used for fixation. For autophagy detection, samples were prepared, fixed and washed as described above. Fixed tissues were dissected in PBS, mounted in Vectashield (Vector Labs, Burlingame, CA) and confocal images were collected on a Zeiss LSM710 confocal microscope and processed with Adobe Photoshop. The following antibodies were used for imaging experiments: rabbit anti-AKH (1:500), rabbit anti-Dilp2 (1:500), rabbit anti-Dilp3 (1:500), mouse anti-Dilp3 (1:500; all gifts of J. Veenstra, Université Bordeaux, Talence, France [34] ), rat anti-Dilp2 (1:500; gift of P. Leopold, Université de Nice, Nice, France [9] ), rabbit anti-AKH (1:500; gift of J. Park, University of Tennessee, Knoxville, TN [8] ). Sugar measurement Haemolymph sugar concentrations were determined as described previously [35] . In brief, 1 μl of haemolymph was obtained from 9–10 L3 larvae and mixed with 9 μl of trehalase buffer (5 mM Tris pH 6.6, 137 mM NaCl, 2.7 mM KCl). After incubation for 5 min at 95 °C and centrifugation for 10 min at 4 °C at 15,000 r.p.m., the supernatant was used for sugar measurement. Glucose (GO) Assay Kit (GAGO-20, Sigma-Aldrich, St Louis MO) was used according to the manufacturer’s instructions to measure glucose. For trehalose measurements, supernatants were first incubated at 37 °C overnight with trehalase (T8778-1UN, Sigma-Aldrich Co. St Louis, MO) and glucose levels were then measured as above. Samples were read in 96-well plates (3641, Corning Life Sciences, Corning NY) at 540 nm using a Victor 3 V 1420 multilabel counter (Perkin Elmer, Waltham MA). mRNA measurement Twenty-five brains per sample were dissected in PBS, and total RNA was isolated using a Direct-zol RNA MiniPrep kit (R2050, Zymo Research, Irvine CA). RevertAid First-Strand cDNA Synthesis Kit (K1621, Thermo Scientific, Pittsburgh PA) was used for reverse transcription of 600 ng of total RNA. Products were amplified by PCR using Ex Taq DNA Polymerase (RR001, Clontech Laboratories, Mountain View CA) for 34 reaction cycles, which was determined in control experiments to be within a linear range of amplification. Primer sequences were as follows: Dilp2-F 5′-CTGAGTATGGTGTGCGAGGA-3′; Dilp2-R 5′-CAGCCAGGGAATTGAGTACAC-3′; Dilp3-F 5′-GACCAAGAGAACTTTGGACCC-3′; Dilp3-R 5′-CAGCACAATATCTCAGCACCTC-3′; Rp49-F 5′-CGGATCGATATGCTAAGCTGT-3′; Rp49-R 5′-GCGCTTGTTCGATCCGTA-3′. How to cite this article : Kim, J. et al. Dietary sugar promotes systemic TOR activation in Drosophila through AKH-dependent selective secretion of Dilp3. Nat. Commun. 6:6846 doi: 10.1038/ncomms7846 (2015).